Chemical potential oscillations from nodal Fermi surface pocket in the underdoped high-temperature superconductor YBa2Cu3O6+x The electronic structure of the normal state of the underdoped cuprates has thus far remained mysterious, with neither the momentum space location nor the charge carrier type of constituent small Fermi surface pockets being resolved. Whereas quantum oscillations have been interpreted in terms of a nodal-antinodal Fermi surface including electrons at the antinodes, photoemission indicates a solely nodal density-of-states at the Fermi level. Here we examine both these possibilities using extended quantum oscillation measurements. Second harmonic quantum oscillations in underdoped YBa 2 Cu 3 O 6+ x are shown to arise chiefly from oscillations in the chemical potential. We show from the relationship between the phase and amplitude of the second harmonic with that of the fundamental quantum oscillations that there exists a single carrier Fermi surface pocket, likely located at the nodal region of the Brillouin zone, with the observed multiple frequencies arising from warping, bilayer splitting and magnetic breakdown. Although high- T c cuprate superconductors have a history spanning a quarter of a century [1] , [2] , quantum oscillations in these materials have only been measured as recently as a few years ago [3] , [4] , [5] , [6] , [7] , [8] , [9] , [10] , [11] , [12] , by employing high magnetic fields to weaken superconductivity. Interestingly, their advent has signalled a re-evaluation of the electronic structure in the normal state of the underdoped cuprates. Where, previously, the very existence of quasiparticles was questioned in the normal state of the underdoped cuprates [13] , quantum oscillations have uncovered quasiparticles consistent with the existence of a Fermi liquid within this regime [8] . Despite the progress made by quantum oscillations that complement a broad array of other experiments in discerning the normal state of the cuprates, fundamental mysteries remain both in interpreting the results of quantum oscillation measurements, and in reconciling them with other experimental techniques. Quantum oscillation results have been interpreted in terms of a nodal-antinodal Fermi surface [4] , [9] , [11] , [12] arising from spatial symmetry breaking, where the antinodal sections correspond to electron pockets [12] , and the nodal sections correspond either to closed hole pockets or open sheets [11] in models proposed thus far. Multiple frequencies can arise not only from closed sections such as these, but also from warping, splitting, and magnetic breakdown effects of a single Fermi surface section. The nodal locations refer to k nodal =[π/2 a , π/2 a ] in the Brillouin zone, and the antinodal locations refer to k antinodal =[π/ a , 0] in the Brillouin zone, where a is the lattice constant. This picture, however, is in direct contrast with the observation made by photoemission experiments of a significant (~50 meV) gap in density-of-states at the Fermi level at the antinodes [14] , [15] , [16] . Against this backdrop of contradictory scenarios, an unambiguous interpretation of quantum oscillation results in terms of momentum space location, charge carrier type, and single or multiple surfaces in the case of the underdoped cuprates has remained elusive [3] , [4] , [5] , [6] , [7] , [8] , [9] , [10] . Quantum oscillations in the case of a fixed chemical potential cannot discern the sign of charge carriers or whether there are single or multiple types of charge carrier present [17] , causing recourse, thus far, to less direct probes such as the Hall effect and thermopower, and calculations of the electronic structure to infer a nodal-antinodal Fermi surface [4] , [9] , [18] , [19] , [20] . In this work, we observe well-defined second harmonic quantum oscillations from a broad array of torque and contactless resistivity experiments performed at the National High Magnetic Field Laboratory in a 45 T DC magnet at temperatures 30 mK T 1.5 K, and in 65 & 85 T pulsed magnets at temperatures 1 K T 5 K, over an angular range 0 θ 60°. The second harmonic is extracted by fitting and subtracting from the data an unconstrained sum of four low frequencies ( F <700T), similar to those earlier reported in references 6 , 7 , 9 , 10 , and a slowly varying aperiodic background (fit procedure shown in Methods). From the analysis of the measured second harmonic oscillations, we present the surprising finding that the harmonic content in underdoped YBa 2 Cu 3 O 6+ x ( x =0.56) arises from oscillations of the chemical potential, which are enhanced compared to normal metals by the quasi-two-dimensional topology of the Fermi surface [17] , [21] , [22] , [23] , [24] . Oscillatory features corresponding to multiple frequencies in 1/ B previously reported [3] , [6] , [7] , [9] are observed: ( F α =535(5) T, F γ 1 =440(10) T, F γ 2 =610(20) T) down to 22 T, and F β =1,550(50) T at the lowest temperatures 1 K (to be presented elsewhere); yet, we conclude, from the magnitude and phase of the second harmonic with respect to the fundamental oscillations, that the Fermi surface consists chiefly of a single carrier pocket, the multiple frequency components arising from effects of finite c -axis dispersion, bilayer splitting, and magnetic breakdown. The next question relates to the location of this quasi-two-dimensional pocket. We consider complementary experiments: photoemission experiments at zero field [14] , [15] , [16] , optical conductivity experiments up to 8 T (refs 25 , 26 ), and high field heat capacity experiments (ref. 27 ) indicate a solely nodal concentration of the density-of-states at the Fermi level. Given that the form of quantum oscillations persist unchanged down to 22 T where the d-wave superconducting gap is well developed, indications are that the observed quasi-two-dimensional Fermi surface pocket is located at the nodal region of the Brillouin zone. Observations of second harmonic oscillations A number of observations relating to the second harmonic reveal departures from the oscillatory behaviour expected from the standard Lifshitz–Kosevich theory that assumes a fixed chemical potential [17] . 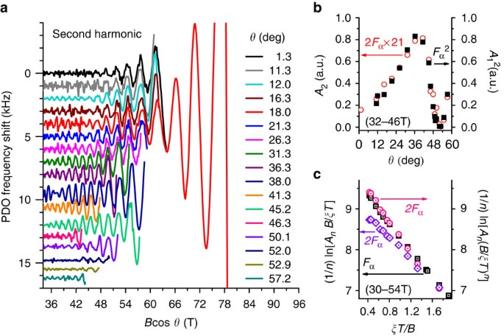Figure 1: Angular and temperature dependence of second harmonic quantum oscillations. (a) Field-dependence of the second harmonic (2F) extracted from the data in ref.28at different anglesθbetween the crystallinec-axis and the magnetic field after having subtracted fits to the fundamental (F) and a slowly varying background (subtraction procedure shown in Methods). The data are plotted versusBcosθto facilitate a comparison of the relative phase. The second harmonic amplitude falls to a small value near 54° (at which the fundamental undergoes a spin zero28), following which it recovers with the same phase at higher angles. (b) A comparison of the Fourier amplitude of the second harmonic obtained over the field interval indicated (red circles) against the rescaled square of the amplitude of the fundamental (F2) (black squares) reveals that they precisely track each other over a broad range of angles, spanning the spin zero in the fundamental near 54°. (c) Temperature dependence of the fundamental (black squares) and second harmonic (coloured squares). We plot (1/n)1n[AnB/ξT] versusξT/B, wherenis the harmonic index,ξ=2π2kBme/ℏe=14.69 T/K, andAnis the measured harmonic amplitude. The slope of this relation is expected to have the valuem*/me, wheremeis the free electron mass, for both the second harmonic and the fundamental (given the division bynon the left axis). We find, however, an unexpectedly low slope of value 1.3(1) for the second harmonic, which is lower than the slopem*/me=1.6(1) measured for the fundamental. On plotting (1/n)1n[An(B/ξT)n] versusξT/Bfor the second harmonic (pink symbols, right axis), however, the slope of the relation agrees with that of the fundamental. The latter implies that the temperature dependence of the second harmonic is given by(whereRT1=X/sinhX~2Xe−XforX=ξTm*/Bme≪1), as expected from the effects of oscillations in the chemical potential29. Figure 1a shows the second harmonic extracted from quantum oscillations measured on YBa 2 Cu 3 O 6+ x at a series of fixed angles θ (between the crystalline c axis and the magnetic field) as a function of the c -axis magnetic field component B cos θ , where B = μ 0 H is the applied magnetic field (up to 85 T in a pulsed field magnet). We find that the second harmonic oscillations retain a constant phase between θ =0° and 57° at fixed B cos θ (ref. 9 ). A remarkable feature in the data is the absence of a zero in amplitude near ~18°, which is expected in the second harmonic if μ is fixed, given the presence of a spin zero in the fundamental at ~54° (ref. 28 ) ( Fig. 1b ). Instead, the second harmonic amplitude falls to zero at exactly the same angle as the fundamental. Figure 1: Angular and temperature dependence of second harmonic quantum oscillations. ( a ) Field-dependence of the second harmonic (2 F ) extracted from the data in ref. 28 at different angles θ between the crystalline c -axis and the magnetic field after having subtracted fits to the fundamental ( F ) and a slowly varying background (subtraction procedure shown in Methods). The data are plotted versus B cos θ to facilitate a comparison of the relative phase. The second harmonic amplitude falls to a small value near 54° (at which the fundamental undergoes a spin zero [28] ), following which it recovers with the same phase at higher angles. ( b ) A comparison of the Fourier amplitude of the second harmonic obtained over the field interval indicated (red circles) against the rescaled square of the amplitude of the fundamental ( F 2 ) (black squares) reveals that they precisely track each other over a broad range of angles, spanning the spin zero in the fundamental near 54°. ( c ) Temperature dependence of the fundamental (black squares) and second harmonic (coloured squares). We plot (1/ n )1n[ A n B/ξT ] versus ξT/B , where n is the harmonic index, ξ =2 π 2 k B m e / ℏ e =14.69 T/K, and A n is the measured harmonic amplitude. The slope of this relation is expected to have the value m */ m e , where m e is the free electron mass, for both the second harmonic and the fundamental (given the division by n on the left axis). We find, however, an unexpectedly low slope of value 1.3(1) for the second harmonic, which is lower than the slope m */ m e =1.6(1) measured for the fundamental. On plotting (1/ n )1n[ A n ( B/ξT ) n ] versus ξT/B for the second harmonic (pink symbols, right axis), however, the slope of the relation agrees with that of the fundamental. The latter implies that the temperature dependence of the second harmonic is given by (where R T 1 = X /sinh X ~2 Xe − X for X = ξTm */ Bm e ≪ 1), as expected from the effects of oscillations in the chemical potential [29] . Full size image Figure 1c compares the T dependence of the fundamental amplitude A 1 , with that of the second harmonic amplitude A 2 on a linear-log plot normally used to infer the appropriate cyclotron mass. These precisely temperature-controlled measurements were performed with the sample in liquid 4 He in a 60 T generator-driven magnet. Quantum oscillations corresponding to a fixed chemical potential are expected to exhibit a second harmonic with a cyclotron mass twice the fundamental cyclotron mass, yet strangely a fit of the second harmonic to the thermal damping factor ( Fig. 1c ) yields a mass that is too low, by about 25%. 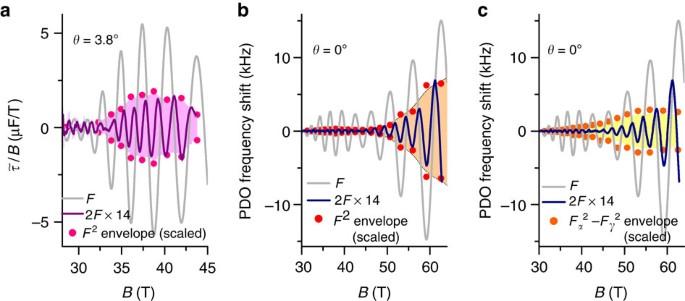Figure 2: Field dependence comparison of second harmonic and squared fundamental quantum oscillations. (a) A comparison of the second harmonic oscillations (thick purple lines) with the scaled square of the amplitude of the fundamental (shown by dots and the envelope shown by shading) versus magnetic field, indicating that they are closely correlated for the oscillatory magnetizationextracted from the magnetic torqueat an angleθ~3.8° measured in the 45 T DC magnet. The dots are extracted from the scaled square of the fundamental oscillations maxima and minima. The actual fundamental oscillations are depicted in light grey. (b) The same repeated for the oscillatory contactless resistivity data atθ~0 measured in the 65T pulsed magnet, showing the same behaviour as ina. (c) A comparison of the second harmonic oscillations (thick navy lines) with the scaled difference between the squared amplitude of the fundamentalαandγcomponents (αandγcomponent fit from ref.9). This would be the expectation for nodalαand antinodalγpockets corresponding to opposite carrier types, we find that the observed second harmonic does not follow this form. Figure 2 shows the detected amplitude of the second harmonic as a function of magnetic field measured using two different methods: magnetic torque in DC fields and contactless resistivity in pulsed fields. The measured second harmonic amplitude is found to accurately scale as the square of the fundamental as a function of magnetic field. This square relationship mirrors that as a function of angle ( Fig. 1b ) and as a function of temperature ( Fig. 1c ). Figure 2: Field dependence comparison of second harmonic and squared fundamental quantum oscillations. ( a ) A comparison of the second harmonic oscillations (thick purple lines) with the scaled square of the amplitude of the fundamental (shown by dots and the envelope shown by shading) versus magnetic field, indicating that they are closely correlated for the oscillatory magnetization extracted from the magnetic torque at an angle θ ~3.8° measured in the 45 T DC magnet. The dots are extracted from the scaled square of the fundamental oscillations maxima and minima. The actual fundamental oscillations are depicted in light grey. ( b ) The same repeated for the oscillatory contactless resistivity data at θ ~0 measured in the 65T pulsed magnet, showing the same behaviour as in a . ( c ) A comparison of the second harmonic oscillations (thick navy lines) with the scaled difference between the squared amplitude of the fundamental α and γ components ( α and γ component fit from ref. 9 ). This would be the expectation for nodal α and antinodal γ pockets corresponding to opposite carrier types, we find that the observed second harmonic does not follow this form. 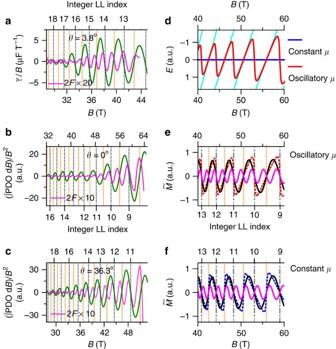Figure 3: Phase relation between second harmonic and fundamental quantum oscillations. (a–c) The fundamental (green) and second harmonic (magenta) extracted from the magnetic torque and integrated contactless resistivity measured in YBa2Cu3O6+xat different field orientationsθas indicated, revealing the same phase behaviour as seen in the schematic figure (e). The magnetization is inferred usingandfrom the magnetic torqueand contactless resistivity, respectively. Integer Landau level filling factors (whenμresides in the gap between two-dimensionalαcomponent Landau levels) are indicated. (d) A schematic showing the Landau level energies (cyan lines) and how the chemical potentialμ(red line) and consequently the magnetization (red line ine) oscillates for a single two-dimensional electron pocket.μjumps between Landau levels (cyan lines) at integer filling factors causing it to be momentarily situated in the Landau gap. (e) The magnetization (red) together with the extracted fundamental (black) and second harmonic (magenta). (f) The corresponding magnetization waveform (blue) when the chemical potential is fixed, giving rise to a second harmonic of opposite sign. Vertical lines in grey correspond to integral Laundau levels, and in orange correspond to half-integral Landau levels. Full size image Waveform of second harmonic oscillations Figure 3 allows us to infer the phase relation between the observed second harmonic oscillations and the fundamental oscillations at 3.8° in the measured torque, 0° in the contactless resistivity signal and at 38° in the contactless resistivity. The second harmonic retains a constant phase with respect to the fundamental, consistent with the sawtooth waveform shown schematically in Figure 3d,e, respectively. This is inconsistent with that expected for quantum oscillations corresponding to a fixed chemical potential, which would lead to a different form (shown in Fig. 3f ) and to a spin zero and phase inversion at 18°, which we do not observe. Figure 3: Phase relation between second harmonic and fundamental quantum oscillations. ( a – c ) The fundamental (green) and second harmonic (magenta) extracted from the magnetic torque and integrated contactless resistivity measured in YBa 2 Cu 3 O 6+ x at different field orientations θ as indicated, revealing the same phase behaviour as seen in the schematic figure ( e ). The magnetization is inferred using and from the magnetic torque and contactless resistivity , respectively. Integer Landau level filling factors (when μ resides in the gap between two-dimensional α component Landau levels) are indicated. ( d ) A schematic showing the Landau level energies (cyan lines) and how the chemical potential μ (red line) and consequently the magnetization (red line in e ) oscillates for a single two-dimensional electron pocket. μ jumps between Landau levels (cyan lines) at integer filling factors causing it to be momentarily situated in the Landau gap. ( e ) The magnetization (red) together with the extracted fundamental (black) and second harmonic (magenta). ( f ) The corresponding magnetization waveform (blue) when the chemical potential is fixed, giving rise to a second harmonic of opposite sign. Vertical lines in grey correspond to integral Laundau levels, and in orange correspond to half-integral Landau levels. 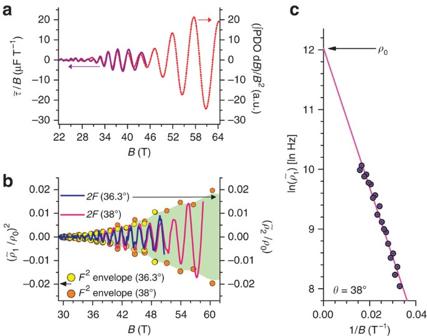Figure 4: Comparison of absolute size of second harmonic and squared fundamental quantum oscillations. (a) Comparison of the magnetizationandinferred from the measured magnetic torque(purple line) and contactless resistivity(red dotted line), respectively. (b) Plot of the second harmonic (atθ~36.3° in fields to 65T and atθ~38° in fields 85 T) divided by the infinite field interceptρ0determined in (c):represented by solid lines is compared withrepresented by solid dots. The ratio of the amplitude of the harmonic (solid lines) to the square of the fundamental (shown by dots and the envelope shown by green shading—extracted from the square of the fundamental oscillations maxima and minima) yields a value of 2Γ38°=1.0(3) from equation (2), from which we obtainΓ38°=0.50(15). (c) Dingle analysis, performed on a linear-log plot of the fundamental oscillations in contactless resistivity (denoted by solid circles, determined from the oscillation maxima and minima after dividing outRT,1) atθ=38° up to fields of 85 T, plotted versus 1/B. The 1/B=0intercept obtained by fitting a straight line (purple) to this plot yieldsρ0=1.6(5)×105Hz in the units of PDO measurements. Full size image Figure 4a shows a collation of quantum oscillations measured in magnetic torque and contactless resistivity, spanning overall a range 22 T–65 T. An identical beat structure previously revealed to correspond to three closely spaced frequencies ( F α =535(5) T, F γ 1 =440(10) T, F γ 2 =610(20) T) is found, confirming the multiple frequency components earlier reported [3] , [6] , [7] , [9] . A significantly higher F β ~1,550(50) T frequency earlier reported [6] is also prominently observed in quantum oscillations measured at the lowest temperatures 1 K (to be presented elsewhere). High sensitivity measurements we report here additionally show that the quantum oscillations with this beat structure persist down to 22 T, where the d-wave superconducting gap is well developed. Figure 4: Comparison of absolute size of second harmonic and squared fundamental quantum oscillations. ( a ) Comparison of the magnetization and inferred from the measured magnetic torque (purple line) and contactless resistivity (red dotted line), respectively. ( b ) Plot of the second harmonic (at θ ~36.3° in fields to 65T and at θ ~38° in fields 85 T) divided by the infinite field intercept ρ 0 determined in ( c ): represented by solid lines is compared with represented by solid dots. The ratio of the amplitude of the harmonic (solid lines) to the square of the fundamental (shown by dots and the envelope shown by green shading—extracted from the square of the fundamental oscillations maxima and minima) yields a value of 2 Γ 38° =1.0(3) from equation (2), from which we obtain Γ 38° =0.50(15). ( c ) Dingle analysis, performed on a linear-log plot of the fundamental oscillations in contactless resistivity (denoted by solid circles, determined from the oscillation maxima and minima after dividing out R T ,1 ) at θ =38° up to fields of 85 T, plotted versus 1/ B . The 1/ B=0 intercept obtained by fitting a straight line (purple) to this plot yields ρ 0 =1.6(5)×10 5 Hz in the units of PDO measurements. Full size image Finally, Figure 4b,c show a comparison between the absolute size of the second harmonic and the square of the fundamental oscillations at an angle where the α oscillations are dominant, both renormalized by the infinite field intercept. These are found to be equivalent in size to within ~30% error. We broadly consider three chief aspects of the experimental data, and understand the unusual behaviour of the second harmonic in terms of the effect of oscillations of the chemical potential μ . Large oscillations in μ tend to occur in layered metals owing to the absence of a large reservoir of phase-incoherent states to pin μ at an essentially constant value [21] , [22] , [23] . Instead of the Landau levels passing through a constant chemical potential—as described in the simplest Lifshitz–Kosevich theory [17] — μ itself oscillates. The chemical potential remains pinned to the highest partially occupied Landau level as its degeneracy changes, jumping from one to the next as the levels become sequentially depopulated on increasing the magnetic field (shown schematically in Fig. 3d ). Oscillations in the magnetization (the de Haas–van Alphen effect) are affected by the jumps in μ , yielding a waveform that resembles a sawtooth (see schematic in Fig. 3e ). We consider the effect that the oscillatory component [mutilde] has on modulating the Onsager phase of the quantum oscillations φ =2 πF / B − η (where the conventional value of η is π ) arising from a two-dimensional pocket giving rise to quantum oscillations of frequency F [17] . The oscillatory magnetization is given by where κ p represents T and B dependent amplitude factors (for example, Dingle, thermal, spin, mosaic spread, etc.) affecting the p th harmonic [17] , and M 0 is the absolute amplitude at infinite field. The effect of chemical potential oscillations are explicitly included in leading order by the expansion of where is the steady part of μ , and [mutilde] is the oscillatory part of μ which is taken to be of the form to leading order [29] . This allows us to rewrite equation (1) in the form where Γ is determined by the relative strength of [mutilde] as discussed below [17] , [29] . While the fundamental frequency continues to be well described by the standard theory for oscillations corresponding to fixed μ , the second harmonic can be dominated by a new contribution of relative weight (see equation (2)) resulting from the oscillations in μ . Here Γ represents the fraction of the total density-of-states at the Fermi level associated with the postulated two-dimensional pocket. In Figure 4a , we compare the fundamental and second harmonic magnetization inferred from the measured torque and from the contactless resistivity (ref. 17 ), where the integration is over the experimental field range. Their similar behaviour and scalability indicates that the oscillations in both quantities have a closely related origin [17] . First, we discuss the phase of the observed second harmonic oscillations. We see that, in the case of strong chemical potential oscillations (where the first term in the prefactor of sin2 φ 0 in equation (2) is dominant), the second harmonic oscillations are in fact out of phase by π from the conventional case of oscillations corresponding to a fixed chemical potential, precisely as we observe in experiment (predictions and comparison with experiment shown in Fig. 3d ). Second, we discuss the amplitude A 2 of the second harmonic, which is expected to vary as the square of the amplitude A 1 of the fundamental in the limit in the case where harmonic enrichment arises mainly from chemical potential oscillations. The experimentally observed square relation as a function of magnetic field at various angles both in the torque and contactless resistivity measurements ( Figs 2 and 4b ) is consistent with this expectation. Also consistent with this expectation is the observed absence of a low-angle spin zero as discussed earlier for the second harmonic ( Fig. 1b ) and the low value of the effective mass inferred from a conventional linear-log plot of the second harmonic, as also mentioned earlier ( Fig. 1c ). Thus far, we have considered a model of a single two-dimensional Fermi surface pocket and hence quantum oscillations with a single periodicity in 1/ B . The predictions of a model including multiple frequencies arising from warping and bilayer splitting of the same pocket are not substantially different from those discussed above (numerical simulations shown in Methods). However, the inclusion of a second two-dimensional Fermi surface pocket associated with carriers of opposite effective charge would lead to an extra harmonic enrichment term from chemical potential oscillations of the opposite sign in addition to the term in equation (2), leading to behaviour in general inconsistent with harmonic components scaling as the square of fundamental components [17] . Figure 2c shows the predicted behaviour for the second harmonic were the α and γ component of the oscillations to be associated with nodal and antinodal pockets, respectively, containing opposite carrier types; this does not fit the experimentally observed form of the second harmonic, ruling out the possibility of the observed quantum oscillations arising from pockets containing opposite carriers. Our finding therefore supports the idea that the observed frequency components are all closely related and are likely to arise from the same two-dimensional pocket, its purely two-dimensional structure modulated by weak warping and bilayer splitting. We next consider what can be learned from the magnitude of the ratio of to A 2 , namely from the magnitude of 2 Γ as defined in equation (2). This ratio is most accurately determined at θ =38° where the γ oscillatory component is weak and the quantum oscillations are dominated by a single periodicity due to the α component [9] , [10] , [28] . In this case Γ ~DOS( α )/(DOS( α )+DOS( γ )+DOS(other)), where 'DOS' stands for density-of-states at the Fermi level and 'other' for any other density-of-states at the Fermi level not associated with the α or γ components. The equivalence in size of and A 2 at θ =38° yields a measured value Γ (38°)=0.50(15) at this angle (see Fig. 4b,c ), from which we estimate an upper bound for DOS(other)/(DOS( α )+DOS( γ )) of about 30%. This suggests that our model of a quasi-two-dimensional Fermi surface pocket giving rise to multiple frequency components α and γ , together with possible magnetic breakdown components, accounts for the majority of the Fermi surface under our experimental conditions in underdoped YBa 2 Cu 3 O 6+ x . The light effective mass ( m *~0.4 m e , yielded by the slope of the dispersion) of an extra open chain Fermi surface observed in photoemission measurements on underdoped YBa 2 Cu 3 O 6+ x would suggest only a small contribution to the density-of-states at the Fermi level. Complementary photoemission experiments at zero field [14] , [15] , [16] , optical conductivity experiments up to 8 T, and high field heat capacity [27] experiments indicate a concentration of density-of-states at the Fermi level solely at the nodal location in momentum space. Taken together with the persistence of quantum oscillations unaltered in form down to low fields ~22 T where the d-wave superconducting gap is well developed, the quasi-two-dimensional Fermi surface pocket that gives rise to multiple frequency components observed by quantum oscillations in underdoped YBa 2 Cu 3 O 6+ x is likely connected with the nodal region of the Brillouin zone. In summary, we find from the form of the second harmonic quantum oscillations in underdoped YBa 2 Cu 3 O 6+ x , that quantum oscillations in this material arise mainly from oscillations of the chemical potential. The phase and magnitude of the second harmonic components relative to the fundamental components allows us to conclude that the Fermi surface consists chiefly of a quasi-two-dimensional pocket giving rise to multiple frequencies, as previously discussed. The Fermi surface pocket responsible for quantum oscillations is likely located at the nodal region, given that these oscillations persist down to low magnetic fields, where the d-wave superconducting gap is well developed, whereas complementary experiments up to these fields [14] , [15] , [16] , [27] find a concentration in the density-of-states at the Fermi level at the nodes of the superconducting wavefunction. Translational symmetry-breaking models proposed thus far are either nodal-antinodal (for example, refs 11 , 12 ), which would be inconsistent with the current experimental results, or comprise solely nodal hole pockets [13] , which would be difficult to reconcile with negative Hall and Seebeck effect [4] , [20] , leaving us with a dilemma. Possible resolutions to this problem involve understanding how a negative Hall and Seebeck effect can arise from a nodal Fermi surface pocket [30] , [31] . Extraction of the second harmonic To isolate the harmonics from the fundamentals, we fit the raw oscillatory signal to a sum of four frequencies of the form where i is the frequency index, A i is the amplitude, Γ i is the damping factor whereas φ i is the phase [17] , [32] . 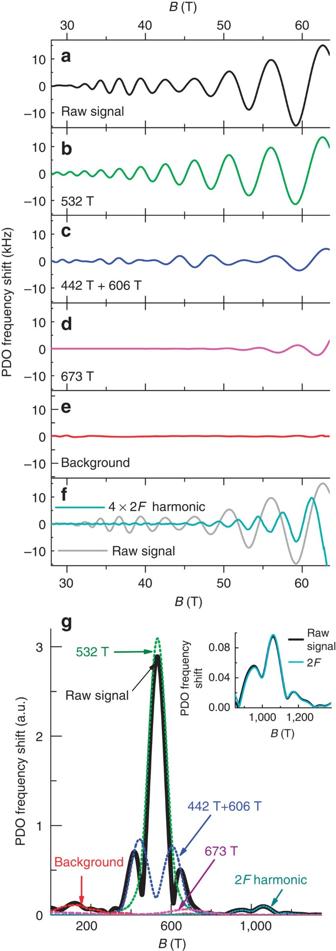Figure 5: Extraction of second harmonic component of the measured quantum oscillation signal. (a) Raw oscillatory signal measured in the contactless resistivity atθ~0 and 1.5 K in the 65 T pulsed magnet. (b–d) Individual frequency components obtained on performing an unconstrained fit to equation (3), similar to those in previous studies6,7,9,10. (e) A slowly varying aperiodic background. (f) The 2Fharmonic in blue (shown inFig. 1bof the main text) is extracted by subtracting components (b–d) from the raw signal, shown in grey. The data and fits are shown over the field range 28≤B≤64T. Fourier transform of each of the components of the measured quantum oscillation signal. (g) Fourier transforms of the contactless resistivity oscillatory data, low frequency (F<700 T) fits, slowly varying background and resulting extracted harmonic component, from panels (a–f), respectively. The inset shows that the Fourier transform of the raw signal and the Fourier transform of the residual 2Fharmonic extracted by subtraction are virtually identical, demonstrating the harmonic content to be unaffected by the subtracted low frequency fits and slowly varying background. Figure 5a shows an example of oscillations in the contactless resistivity, Figure 5b–d show the fit oscillation frequencies, which are similar to those reported in previous experiments [7] , [9] , [10] . The harmonics (shown in Fig. 5f ) are consequently obtained by subtracting the fits plus a small, slowly varying aperiodic background from the raw oscillatory signal (shown in Fig. 5e ). Figure 5: Extraction of second harmonic component of the measured quantum oscillation signal. ( a ) Raw oscillatory signal measured in the contactless resistivity at θ ~0 and 1.5 K in the 65 T pulsed magnet. ( b – d ) Individual frequency components obtained on performing an unconstrained fit to equation (3), similar to those in previous studies [6] , [7] , [9] , [10] . ( e ) A slowly varying aperiodic background. ( f ) The 2 F harmonic in blue (shown in Fig. 1b of the main text) is extracted by subtracting components ( b – d ) from the raw signal, shown in grey. The data and fits are shown over the field range 28≤ B ≤64T. Fourier transform of each of the components of the measured quantum oscillation signal. ( g ) Fourier transforms of the contactless resistivity oscillatory data, low frequency ( F <700 T) fits, slowly varying background and resulting extracted harmonic component, from panels ( a – f ), respectively. The inset shows that the Fourier transform of the raw signal and the Fourier transform of the residual 2 F harmonic extracted by subtraction are virtually identical, demonstrating the harmonic content to be unaffected by the subtracted low frequency fits and slowly varying background. Full size image Figure 5g shows the Fourier transform of each of the individual signal components: it can be seen that the subtracted oscillatory fits and slowly varying background contain only low-frequency features, whereas the inset shows that the remaining 2 F harmonic component after subtraction is identical to that in the raw oscillatory signal. The harmonic content is thus demonstrated to be unaltered by the fit and subtraction process. The extracted harmonic signal is similar to that reported in contactless resistivity [9] , magnetic torque performed in pulsed [7] and DC fields [6] , and c -axis conductivity experiments. In the present magnetic torque experiments, the harmonics are further verified to be independent of the thickness of the cantilever, with measurements on two different cantilevers with thicknesses differing by a factor of 5, yielding the same relative size of harmonics, confirming them to be intrinsic to the sample. Open chain sheets In addition to the sections of Fermi surface originating from the CuO planes, angle resolved photoemission spectroscopy measurements [16] indicate extra bands originating from the BaO orbitals (hybridized with the chains) and from the CuO chains. Whereas the former is situated ~0.5 eV below the Fermi energy [16] , the latter gives rise to open sheets with an effective mass of ~ 0.4 m e . The existence of such a section within the bulk at low temperatures is expected to have a small contribution to the density-of-states at the Fermi level. Numerical simulations Chemical potential oscillations for a quasi-two dimensional Fermi surface including effects of warping can be shown to be similar to the two-dimensional Fermi surface discussed in the main text, using numerical simulations. Numerical simulations of the magnetization (modelled using the method in ref. 22 ) were made for a Fermi surface with multiple components. Fermi surface parameters are taken from ref. 9 , chosen to generate a waveform resembling that observed experimentally. For simulations in which the chemical potential is allowed to oscillate and the carrier density is fixed (that is, N =const. ), the density of electronic states as a function of energy g ( ɛ ) is computed at each value of the magnetic field, with the chemical potential μ determined by the condition (where f ( μ – ɛ ) is the Fermi-Dirac distribution function). The magnetization is calculated from the derivative M =−∂(Ω+ μN )/∂ B | N,T of the Helmholtz free energy Ω+ μN , where is the grand potential. 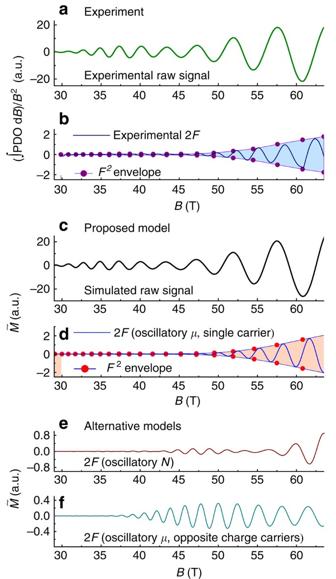Figure 6: Numerically simulated second harmonic oscillations compared with experiment for various scenarios. (a,b) show the experimentally observed raw oscillatory signal and extracted 2Fharmonic in the integrated contactless resistivity. The shaded blue region in (b) is the scaled amplitude envelope ofF2(extracted from the square of the fundamental oscillations maxima and minima) and is found to agree well with the 2Famplitude. (c) Numerical simulations of the oscillatory magnetization signal for a Fermi surface modelled by frequenciesFα=531 T andFγ=532 T, warpings ΔFα=7 T and ΔFγ=72 T, and effective massesafter reference9. The temperature is set toT=1.5 K while the damping factors set to beΓα=140 T andΓγ=120 T. (d) Simulated 2Fharmonic oscillations for the case where the Fermi surface comprises a single carrier pocket with componentsαandγ, yielding oscillations in chemical potential. In this case, the amplitude envelope of the 2Foscillations tracks theF2amplitude envelope (shaded-red region), similar to the case of a single two-dimensional pocket, discussed in the main text. (e) Simulated 2Fharmonic oscillations for the case where the chemical potential is fixed, such that oscillations arise in the carrier density. (f) Simulated 2Fharmonic oscillations for the case where the Fermi surface is nodal-antinodal, comprising nodalαand antinodalγpockets of the same topology but opposite charge carriers, yielding oscillations in chemical potential. The experimental 2Foscillations (shown in (b)) agree in phase and form of amplitude envelope with only one of the simulated cases, that of chemical potential oscillations from a single carrier pocket, shown in (d). Different scenarios are modelled in Figure 6 : first. a Fermi surface with a single carrier pocket with components α and γ from warping, where the oscillations are in chemical potential; second, a Fermi surface with a fixed chemical potential, where oscillations arise from the carrier density; and third, a nodal-antinodal Fermi surface, comprising nodal α and antinodal γ pockets of the same topology but opposite charge carriers, such that the oscillations are in chemical potential. We see that, in the first case, both the phase and amplitude envelope (proportional to F 2 ) of the simulated 2 F harmonic oscillations closely resemble the experimentally observed 2 F harmonic oscillations. In the second case, the phase of the simulated 2 F harmonic oscillations is π out of phase with the observed oscillations, and their amplitude envelope has a form other than F 2 , contrary to experiment. In the third case, whereas the simulated 2 F harmonic oscillations have the same phase as the experimental observation, their amplitude envelope does not have the same form as experiment. Numerical simulations therefore confirm that quantum oscillations in underdoped YBa 2 Cu 3 O 6+ x are consistent with a warped single carrier pocket (simulated in the first case). Figure 6: Numerically simulated second harmonic oscillations compared with experiment for various scenarios. ( a , b ) show the experimentally observed raw oscillatory signal and extracted 2 F harmonic in the integrated contactless resistivity. The shaded blue region in ( b ) is the scaled amplitude envelope of F 2 (extracted from the square of the fundamental oscillations maxima and minima) and is found to agree well with the 2 F amplitude. ( c ) Numerical simulations of the oscillatory magnetization signal for a Fermi surface modelled by frequencies F α =531 T and F γ =532 T, warpings Δ F α =7 T and Δ F γ =72 T, and effective masses after reference 9 . The temperature is set to T =1.5 K while the damping factors set to be Γ α =140 T and Γ γ =120 T. ( d ) Simulated 2 F harmonic oscillations for the case where the Fermi surface comprises a single carrier pocket with components α and γ , yielding oscillations in chemical potential. In this case, the amplitude envelope of the 2 F oscillations tracks the F 2 amplitude envelope (shaded-red region), similar to the case of a single two-dimensional pocket, discussed in the main text. ( e ) Simulated 2 F harmonic oscillations for the case where the chemical potential is fixed, such that oscillations arise in the carrier density. ( f ) Simulated 2 F harmonic oscillations for the case where the Fermi surface is nodal-antinodal, comprising nodal α and antinodal γ pockets of the same topology but opposite charge carriers, yielding oscillations in chemical potential. The experimental 2 F oscillations (shown in ( b )) agree in phase and form of amplitude envelope with only one of the simulated cases, that of chemical potential oscillations from a single carrier pocket, shown in ( d ). Full size image How to cite this article: Sebastian, S. E. et al . Chemical potential oscillations from nodal Fermi surface pocket in the underdoped high-temperature superconductor YBa 2 Cu 3 O 6+ x . Nat. Commun. 2:471 doi: 10.1038/ncomms1468 (2011).